Anisotropic energy flow and allosteric ligand binding in albumin Allosteric interactions in proteins generally involve propagation of local structural changes through the protein to a remote site. Anisotropic energy transport is thought to couple the remote sites, but the nature of this process is poorly understood. Here, we report the relationship between energy flow through the structure of bovine serum albumin and allosteric interactions between remote ligand binding sites of the protein. Ultrafast infrared spectroscopy is used to probe the flow of energy through the protein backbone following excitation of a heater dye, a metalloporphyrin or malachite green, bound to different binding sites in the protein. We observe ballistic and anisotropic energy flow through the protein structure following input of thermal energy into the flexible ligand binding sites, without local heating of the rigid helix bundles that connect these sites. This efficient energy transport mechanism enables the allosteric propagation of binding energy through the connecting helix structures. Allosteric interactions between remote sites in a protein structure play an important role in many biological processes. For example, the binding of an effector molecule at a distant site modulates ligand binding affinity and the activity of many enzymes. Phenomenological models have been developed that successfully describe the thermodynamics of allostery but do not reveal its underlying molecular mechanism. The structure-based view of allostery postulates a series of structural changes or pathways of structural distortion between the two sites that are usually inferred from the equilibrium structures of the two end states [1] , [2] . More recent models of allostery focus on changes in the energy landscape induced by ligand binding that lead to population shifts and changes in protein conformational dynamics [3] . In either view, the role of dynamics is critical in moving free energy from one part of the structure to the other. Several groups have postulated that energy flow through specific pathways is required for proteins to direct energy in useful ways, for example, in allosteric ligand binding [4] , [5] , [6] , [7] , [8] . Such energy transport pathways are thought to couple the energy released in a binding event to a distant target structure, to achieve a functional structural change [9] . Energy transport in a protein may proceed by intramolecular vibrational energy transfer through local protein structures [10] , [11] . It is also possible that efficient energy flow occurs through collective (phonon-like) motions of the protein structure [12] , [13] . Physical models have been developed that describe the dynamics of energy flow in terms of the protein structure and vibrational modes [14] , [15] . Molecular dynamic (MD) simulations have been particularly useful for identifying specific structures involved in energy transport [7] , [16] , [17] , [18] . For example, MD calculations have identified energy transport channels in PDZ domains thought to be relevant for intramolecular signalling between remote sites in the protein structure [7] . Experimental evidence exists for anisotropic cooling pathways in haem proteins subsequent to photoexcitation of the haem, which deposits a large amount of excess energy in the interior of the protein [13] , [19] , [20] , [21] , [22] . Both theory and experiment indicate that energy flow pathways are sensitive to the protein structure and dynamics, but there is no clear relationship between energy transport mechanisms and allosteric coupling between remote sites of a protein structure. Femtosecond pump-probe spectroscopy methods are required to measure the ultrafast flow of energy through a protein structure. The approach is straightforward in concept: an ultrafast (~30 fs) visible laser pulse is absorbed by a heater dye bound to the protein, and is then converted to vibrational energy through rapid internal conversion. The ‘hot’ ground state of the heater dye then cools by transferring energy to the protein, and ultimately that heat flows through the protein and out to the solvent. Ultrafast time-resolved infrared (TRIR) spectroscopy is used to track the dynamics of the protein and solvent heating, since the spectra of both are sensitive to temperature, a property that we have exploited in extensive studies of protein folding dynamics using a laser-induced T-jump [23] , [24] . Similar methods have been developed by the Hamm group to study energy flow through peptides [25] , [26] , [27] , and energy flow from solvent into myoglobin detected by the response of a CO molecule trapped within a binding pocket [28] . These experiments provide a direct measure of the dynamics of energy transport through the protein structure. The transient IR spectrum provides information about the anisotropy of the energy flow, through transient changes in specific backbone amide or side chain vibrations [26] , [29] , [30] , [31] . Here, we study the connection between allosteric ligand binding in bovine serum albumin (BSA) and anisotropic energy flow, using a metalloporphyrin (MP) or malachite green (MG) as a heater dye. Albumin, the major protein component in serum, is important in a wide range of functions including metabolism, pharmacokinetics and elimination of toxins [32] . Albumin acts as a carrier protein with an amazing capacity for binding a wide range of ligands from fatty acids to haem and drugs such as ibuprofen and warfarin. It consists of multiple globular domains that are capable of binding ligands cooperatively, analogous to allosteric binding observed in multimeric proteins. Allosteric modulation of ligand binding to sites in the different domains is observed with fatty acid binding to multiple sites in the protein [33] . Metalloporphyrin binds to the FAI site in subdomain IB [34] , [35] , whereas MG normally binds to Sudlow site I in subdomain IIA based on site marker competition experiments [36] . These sites are allosterically linked, such that binding of a ligand at one site changes the binding constant at the other by about an order of magnitude [34] . Visible light excitation of MP or MG bound to the protein results in rapid energy flow to the protein due to internal conversion and subsequent relaxation processes [37] . The dynamics of energy flow through the secondary structure of BSA was probed using ultrafast time-resolved infrared spectroscopy [37] , [38] . We observe anisotropic energy flow through the protein structure following input of thermal energy into the flexible ligand binding sites, without local heating of the rigid helix bundles that connect these sites. This efficient energy transport mechanism enables the allosteric propagation of binding energy through the connecting helix structures. Binding of heater dyes to BSA The first requirement for the heat transport experiments is to bind the heater dye, either Cu(II) meso-tetra(4-sulfonatophenyl)phorphine (MP) or malachite green (MG), to a specific site within the protein. We characterized the interaction of each heater dye with the protein using UV–vis absorbance spectroscopy as shown in Fig. 1 . Both heater dyes exhibit changes in their absorbance spectra that are characteristic of binding to hydrophobic binding sites in the protein. The Soret band of the MP in aqueous solution is centred at 399 nm, but shifts to 420 nm when bound to the protein ( Fig. 1a ). The porphyrin binding site in albumin is a D-shaped cavity (fatty acid binding site I, FAI) that is lined by hydrophobic sidechains of subunit IB. Similar spectral shifts have been observed for binding of haem to FAI [39] , consistent with binding of the Cu porphyrin to the same site. MG in water has a doublet centred at 595 nm (black trace in Fig. 1b ), characteristic of dimer formation due to π-stacking of the phenyl rings, which causes exciton splitting of the lowest energy π–π* transition. Titration of a solution of MG dimers with BSA causes the exciton doublet to collapse to a single, red-shifted band at 628 nm (red trace in Fig. 1b ). These data are consistent with the breakup of the dimer due to binding of MG to a site within BSA. The monomer peak is red-shifted by 10 nm compared with the monomer peak of MG in aqueous solution (at 1 μM), indicating it is bound in a hydrophobic site. Competitive site marker experiments previously concluded that the MG is bound to Sudlow site I in subdomain IIA (FA7) of BSA [36] . The present results confirm that both MP and MG bind to hydrophobic binding sites within the protein, in subdomains I and II respectively [40] . 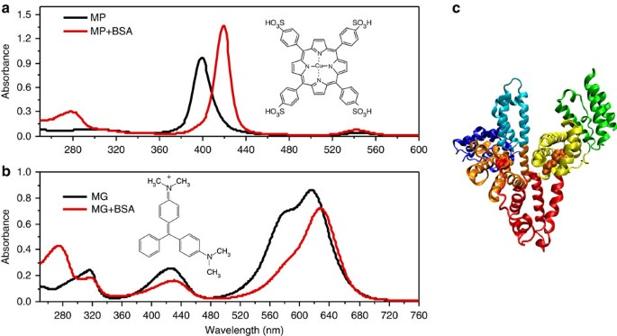Figure 1: UV–vis absorbance spectra of heater dye binding to albumin. (a) 1 mM metalloporphyrin (MP) and (b) 2 mM malachite green (MG) without added bovine serum albumin (BSA; black) and with 1 mM BSA in 50 mM phosphate buffer (red); (c) structure of human serum albumin (Protein Data Bank 1O9X) with myristate bound to Sudlow site I in subunit IIA (red spheres) and site II in subunit IIIA (orange spheres). Figure 1: UV–vis absorbance spectra of heater dye binding to albumin. ( a ) 1 mM metalloporphyrin (MP) and ( b ) 2 mM malachite green (MG) without added bovine serum albumin (BSA; black) and with 1 mM BSA in 50 mM phosphate buffer (red); ( c ) structure of human serum albumin (Protein Data Bank 1O9X) with myristate bound to Sudlow site I in subunit IIA (red spheres) and site II in subunit IIIA (orange spheres). Full size image Ultrafast infrared BSA heating signature The IR spectral response of ultrafast BSA heating was determined using a 30 fs visible laser pulse to locally heat the bound MG dye. The 800 ps time-resolved infrared (TRIR) spectrum of the binary MG/BSA complex is compared with that of free MG in Fig. 2b . On this timescale, most of the dye molecules have relaxed back to the ground state, except for a small population of the long-lived triplet state that contributes two weak bands at 1,617 and 1,588 cm −1 to the MG spectrum. In contrast, the MG/BSA complex has two additional bands at 1,622 and 1,676 cm −1 that we attribute to heating of the protein. These features grow in with a lifetime of 40 ps and persist for as long as we can measure in the ultrafast experiment (about 1 ns). Since these bands are missing in the free MG transient spectrum, they are clearly due to the protein complex. On this timescale, the heat initially deposited in the MG should be completely equilibrated with the protein structure due to vibrational energy transfer processes, which are expected to occur within tens of picoseconds. The protein amide I mode dominates this spectral region, with distinct contributions from the different secondary structural components of the protein backbone. Transient heating of a protein solution is known to cause shifts in the amide I band due to anharmonic coupling with low frequency modes that are vibrationally excited by the increasing temperature [27] . We conclude that the transient amide I features are due to heating of the protein by vibrational energy transfer from the MG heater dye. This conclusion is supported by the ultrafast rise of the heating signal (1 ps, as shown below), similar to what has been observed by the Hamm group for heating of the PDZ protein structure by photo-isomerization of an azobenzene trigger [41] . Photo-driven protein conformational changes are generally slower, such as the conformational change in myoglobin driven by CO photolysis from the haem, which takes about 50 ps (ref. 42 ). 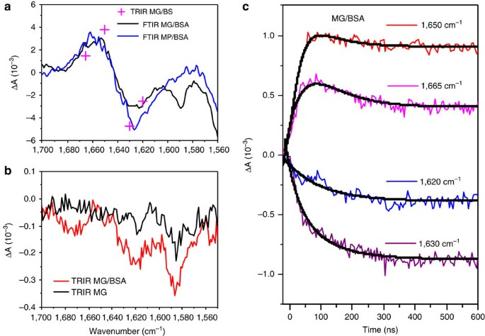Figure 2: IR spectral signature of albumin heating. (a) Equilibrium temperature dependent Fourier transform infrared (FTIR) difference spectra of 800 μM malachite green/BSA (MG/BSA) and metalloporphyrin/BSA (MP/BSA) (25–20 °C) with 300 ns transient IR amplitudes overlaid as magenta crosses (scaled to match ΔT of FTIR difference spectrum); (b) 800 ps TRIR spectrum of free MG (black) and the MG/BSA complex (red), obtained as an average of 2,000 laser pulses; (c) ns T-jump transients of the MG/BSA complex monitored at the indicated frequencies, showing the timescale for development of equilibrium difference features (average of 1,000 shots). Figure 2: IR spectral signature of albumin heating. ( a ) Equilibrium temperature dependent Fourier transform infrared (FTIR) difference spectra of 800 μM malachite green/BSA (MG/BSA) and metalloporphyrin/BSA (MP/BSA) (25–20 °C) with 300 ns transient IR amplitudes overlaid as magenta crosses (scaled to match ΔT of FTIR difference spectrum); ( b ) 800 ps TRIR spectrum of free MG (black) and the MG/BSA complex (red), obtained as an average of 2,000 laser pulses; ( c ) ns T-jump transients of the MG/BSA complex monitored at the indicated frequencies, showing the timescale for development of equilibrium difference features (average of 1,000 shots). Full size image We previously characterized the excited state dynamics of MG and found that it undergoes ultrafast internal conversion to the ground state (GS) at a conical intersection accessed from a twisted intramolecular charge transfer (TICT) state [37] , followed by vibrational relaxation of the GS within 8 ps. When bound to the protein, the internal conversion dynamics is slowed slightly, likely because of hindered rotation of the dimethylamino group and the reduced dielectric of the protein environment, both of which slow the TICT process leading to slower internal conversion and slower energy release from the heater dye. Thus, the MG 1,588 cm −1 bleach recovery lifetime of 43±2 ps observed for the MG/BSA complex represents the bound MG excited state lifetime and not the time required to transfer heat to the protein. The rise time of the protein heating signal is 40±8 ps, synchronous with the recovery of the MG bleach signal, as expected for direct energy transfer from the heater dye to the protein. Since the TICT process is rate limiting, this experiment does not resolve the heat flow dynamics; nevertheless it does characterize the amide I signature of ultrafast protein heating. Figure 2 also compares the 800 ps TRIR spectrum with the equilibrium temperature-dependent FTIR difference spectra of the MG/BSA and MP/BSA complexes, obtained by subtracting the spectrum at 20 °C from that at 25 °C. There are clear differences between the equilibrium FTIR spectrum and the ultrafast IR spectrum. The contrast between the equilibrium and transient spectra is not due to a difference in magnitude of the temperature change between the two experiments, since we estimate that the transient temperature increase produced by the heater dye is about 5 °C, assuming the energy of the 550 nm photon (3.6 × 10 −19 J) absorbed by MG is thermalized into a spherical volume of r =2 nm (the approximate size of subdomains I and II) and using the density and specific heat capacity of BSA ( ρ =1.35 g cm −3 and C p =1.5 J g −1 °C). Furthermore, the FTIR difference features are unchanged as the temperature is increased over the range of ΔT=5–25 °C, except that their amplitudes increase monotonically. The FTIR difference spectrum reveals shifts in several subcomponents of the amide I band, with the biggest change due to the solvated helix band at 1,630 cm −1 , as expected for the predominantly helical structure of BSA [40] , [43] . The solvated helix band broadens and shifts with increasing temperature, producing the characteristic derivative shaped feature in the difference spectrum. Previous work by our group demonstrated that similar changes to the solvated helix band of several model proteins are due to perturbation of the helix structure due to solvent rearrangement around the helix backbone [44] . On some longer timescale, the ultrafast IR spectrum must evolve into the equilibrium spectrum. This timescale was determined by nanosecond T-jump experiments, shown in Fig. 2c . The MG was heated with a 10 ns visible pulse, and the protein response was monitored at IR probe frequencies corresponding to the key features in the FTIR difference spectrum. The amplitudes of the transient IR absorbance at 300 ns are overlaid on the equilibrium FTIR difference spectrum in Fig. 2a , showing good agreement with one another. Thus, the ultrafast IR spectrum represents the heating signature before the structural changes detected in the equilibrium FTIR spectra because the latter occur on the nanosecond timescale. Finally, the amide I transient absorbance features due to the structural changes persist for several milliseconds, which is the time required for the heat to diffuse out of the excited volume [45] . These results demonstrate a clear separation in time between the initial heating process and subsequent structural changes, meaning that it should be possible to follow the heat flow dynamics using the amide I spectral heating signature and a heater dye with faster internal conversion dynamics. Heat flow dynamics and allostery in BSA The heat transfer dynamics was resolved in experiments with the metalloporphyrin (MP) heater dye as shown in Fig. 3 . Without the protein, the MP excited state decays within ~700 fs by internal conversion, followed by relaxation of the hot ground state through vibrational energy transfer to the water. There are no strong porphyrin bands in this region, so we assign the broad, featureless transient absorbance observed for free MP ( Fig. 3a , black traces) to heating of the D 2 O solvent based on the close match with the temperature dependent FTIR difference spectrum of D 2 O. In contrast, the transient IR spectra of the MP/BSA complex (blue traces) have several bands that are not present in the spectrum of the MP alone and are thus attributed to the protein. The transient IR spectrum of MP/BSA evolves with time (from 2.5–138 ps in Fig. 3a ), as the distinct initial heating pattern converts to the fully equilibrated spectrum at longer times. Furthermore, the long time (>100 ps) MP/BSA spectrum is essentially identical to the MG/BSA spectrum ( Fig. 2b ), which also represents the fully equilibrated, isotropic heating signature. Regardless of which ligand binding site is heated, the same global heating profile is produced within 100 ps. Therefore, we conclude that deposition of heat in either site results in rapid global heating of the protein, yielding the same net heating profile. 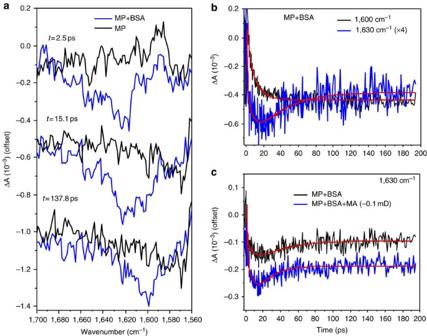Figure 3: Anisotropic heat flow in the MP/BSA complex. (a) Ultrafast IR spectra of the free MP (black) and the MP/BSA complex (blue) at the indicated delay times; (b) IR transients for the MP/BSA complex monitored at 1,600 cm−1(black), which probes the D2O solvent response and at 1,630 cm−1(blue), which probes the protein backbone response; (c) comparison of the IR transients for the MP/BSA with and without sodium myristate. Spectra and transients are obtained from an average of 2,000 laser pulses. Figure 3: Anisotropic heat flow in the MP/BSA complex. ( a ) Ultrafast IR spectra of the free MP (black) and the MP/BSA complex (blue) at the indicated delay times; ( b ) IR transients for the MP/BSA complex monitored at 1,600 cm −1 (black), which probes the D 2 O solvent response and at 1,630 cm −1 (blue), which probes the protein backbone response; ( c ) comparison of the IR transients for the MP/BSA with and without sodium myristate. Spectra and transients are obtained from an average of 2,000 laser pulses. Full size image The initial heat flow process through the protein is anisotropic, since the transient IR spectrum at early times (2.5–30 ps) is distinct from the isotropically heated protein signature observed at longer delay times ( t >100 ps). The kinetics provides additional evidence for anisotropic heat flow ( Fig. 3b ). The kinetics monitored at 1,600 cm −1 is dominated by the D 2 O response, whereas the maximum of the protein response is at 1,630 cm −1 , so these two probe frequencies independently monitor heating of the solvent and the protein. In the absence of the protein, the 1,600 cm −1 D 2 O heating signal produced by excitation of free MP is fit by a single exponential function with a lifetime of 10 ps, which represents the lifetime for equilibration of the hot MP ground state with the surrounding solvent. For MP bound inside the protein, the 1,600 cm −1 D 2 O response is dominated by a fast phase with the same lifetime of 10 ps and a small amplitude slower phase (black trace, Fig. 3b ). The protein transient bleach at 1,630 cm −1 exhibits a fast (1 ps) rise, followed by a decay consisting of two exponential phases of nearly equal amplitudes and lifetimes of 10 and 29 ps (blue trace, Fig. 3b ). The fast rise represents the initial heating of the protein structure, which occurs significantly faster than the vibrational energy transfer to solvent in free MP. Low frequency porphyrin vibrations such as doming and ruffling modes are known to strongly couple to the protein structure in the case of haem proteins, which could facilitate ultrafast energy transfer [46] . The decay of the protein signal represents equilibration of the initial anisotropic heat distribution in the protein with the surrounding structure and with the solvent. The 10 ps decay phase is congruent with the primary phase of the water heating by the bound MP and also matches the timescale for direct vibrational energy transfer from the free MP to water. The timescale of this phase is much faster than what is predicted for diffusive heat flow through the protein structure [14] . The 10 ps phase also has a spectral signature that is distinct from the isotropic heating signature. Therefore, we interpret this phase as ballistic, anisotropic heat flow that couples energy through a direct pathway out to the surrounding water. Since this ballistic phase has the same lifetime as direct vibrational energy transfer from free MP to water, it is likely that the energy transfer step from the protein to solvent is rate determining in this case, such that the actual rate of ballistic heat transport is not resolved. The slower (29 ps) decay phase is the lifetime expected for diffusive heat flow through the protein structure [47] . The initial anisotropic heating spectrum is converted to the fully equilibrated spectrum on this timescale, consistent with diffusion of the heat through the entire protein structure. The connection between allostery and ballistic heat flow through the protein structure is established by comparing the kinetics of this process with and without the allosteric effector sodium myristate. Myristate binding to the high affinity FA2 site is known to change the binding affinity of metalloporphyrins to the FA1 site [34] . Figure 3c compares the kinetics of heat flow through the protein with and without myristate, monitored at 1,630 cm −1 . Without myristate, the decay of the initial protein heating signature occurs in two phases (ballistic and diffusive) of nearly equal amplitude, but, when the fatty acid is bound to the FA2 site, the decay is dominated (75%) by the ballistic (10 ps) component. The link between the porphyrin and fatty acid binding sites in subdomains I and II was previously established by studies that showed binding of a ligand to either site perturbs the structure and binding affinity of the other [34] . Our results demonstrate that the coupling between these sites also impacts the heat flow through the protein structure. Binding of the allosteric effector results in a significant increase in the efficiency of ballistic, anisotropic heat flow through the protein. The observation of anisotropic, ballistic energy flow in BSA is related to the mechanism of propagation of local structural changes to remote sites within the protein structure, as required for allosteric ligand binding. We postulate that efficient energy transport between the flexible ligand binding sites is made possible by the connecting rigid helix bundles. The A and B subdomains consist of six and four helix bundles, respectively, pinned together by multiple disulphide bonds that confer stability and rigidity. Residues from both the flexible loop regions and the more rigid helix bundles form the MP and MG binding sites, in subdomains IB and IIA, respectively. Evidence from crystal structures [34] reveals that a conformational transition driven by myristate binding to HSA causes a 16° rotation of domains I and III with respect to domain II. The connecting extended loop structures are flexible enough to allow this rotation, whereas the helix bundles move as rigid units. Reorientation of the helix bundles forms a new binding site (FA2) and modifies the other sites as well, in part by perturbing the size of the binding pockets. This conformational transition modulates the ligand binding affinity of the drug sites as well as the haem site [34] . We emphasize that this mechanism is inferred from crystal structures of the protein with and without bound ligand, which do not provide direct evidence for dynamic long-range interaction of the flexible ligand binding sites with one another through the rigid helix bundles. We have shown that input of thermal energy into the porphyrin (FAI) site results in ballistic energy flow through the protein structure. The efficiency of this ballistic heat flow depends on the allosteric interaction of the FAI site with the drug binding site (FAII). Energy flow between these sites might be expected to heat the intervening rigid helix bundles that connect subdomains IB and IIA. These connecting helices give rise to the dominant 1,650 cm −1 buried helix band in the FTIR spectrum of BSA, but this band is conspicuously absent in the ultrafast IR heating spectrum. We conclude that the ballistic heat flow occurs without local heating of the helix bundles. There is some precedent for propagating the energy of local structural rearrangements across a protein structure through rigid helical domains. For example, the structural transition of myoglobin induced by ligand photodissociation from the haem involves movement of the helices as rigid bodies and relaxation of the more flexible connecting turns [42] . Previous work by the Hamm group showed that the mechanism of energy transport through a helical peptide model depends on its flexibility. Below 270 K, the peptide model is rigid and ballistic heat flow occurs through collective motions of the helix backbone. In contrast, above this temperature the backbone becomes more flexible, and energy transport occurs through intramolecular vibrational relaxation (IVR), a diffusive process that occurs through localized vibrational modes (local heating). Our results show that energy can move through the rigid helix bundles of BSA using the former mechanism, by exciting collective motions of these structures, without local heating of the helices. While such collective motions might also involve the side chains, the helical backbone provides a direct structural connection between the two ligand binding sites. In effect, local heating of the flexible ligand binding sites causes perturbations that are transmitted through the helix bundles, which act as rigid rods that connect the flexible regions and so efficiently transport energy through the protein structure. Therefore, the observation of anisotropic energy flow through the BSA structure supports the proposed mechanism for the allosteric transition. We postulate that this type of anisotropic energy flow through a protein structure is a general allosteric mechanism for the transport of local binding energy to remote sites in proteins. Sample preparation Malachite green (MG, Alfa Aesar) and Cu(II) meso-tetra(4-sulfonatophenyl) phorphine (MP, Frontier Scientific) were used as received. Their chemical structures are shown in Fig. 1 . Bovine serum albumin (98%, essentially fatty acid free, essentially globulin free) was purchased from Sigma-Aldrich. 50 mM phosphate buffer solution (pH=7.0) was prepared from potassium phosphate monobasic (KH 2 PO 4 , A.C.S. reagent) and potassium phosphate dibasic (K 2 HPO 4 , A.C.S. reagent) in a 1:1 ratio in D 2 O (99.9% D, Cambridge Isotope Laboratories). Potassium deuteroxide (KOD, 40% wt. % solution in D 2 O 98+ atom %D, Sigma-Aldrich) and deuterium chloride solutions (35 wt. % in D 2 O, 99 atom % D, Sigma-Aldrich) were used for pH adjustment of the buffer. MG, MP and BSA were dissolved in the 50 mM phosphate buffer (pH=6.0) for FTIR, UV–vis and TRIR measurements. Time-resolved infrared spectroscopy Nanosecond T-jump IR measurements were made using well-established methods developed in our laboratory [41] . Ultrafast infrared measurements were made using a femtosecond pump-probe technique. The TRIR system was designed in the following way: 800 nm laser pulses (1 kHz repetition rate, 30 fs pulse width) were generated in a femtosecond Ti:sapphire regenerative amplifier (Legend Elite, Coherent) seeded by a femtosecond Ti:sapphire mode-locked oscillator (Mantis, Coherent). The Legend output power of 3.6 W was split in a 1:1 ratio and sent into two OPA systems (OPerA Solo, Coherent) used to generate UV–vis pump and IR probe laser pulses, respectively. The 550 nm excitation wavelength was generated by frequency doubling the OPA signal beam. The pump beam was delayed by a computer controlled translation stage (Newmark System). The infrared beam was produced by difference frequency generation in a AgGaS crystal, then split into probe and reference beams by a CaF 2 beamsplitter (50/50±10% R/T, 2–8 μm, ISP Optics). The IR probe and reference beams pass through the sample and then are dispersed in a ¼ m spectrograph and detected by an ImagIR infrared camera (HgCdTe, 2–10 μm, 128 × 128, Santa Barbara Focalplane). The 550 nm pump beam (2.5 mW) is focused on the sample and overlaps with IR probe beam. The relative polarization between the pump and probe beams is set at the magic angle (54.7°). An optical chopper (3501, New Focus) is used to modulate the excitation beam at 500 Hz to obtain the transient absorbance signal. The sample solution is flowed using a fluid metering RHSY lab pump (Scientific Support) through a demountable liquid flow cell with swagelok fittings (DSC-S25, Harrick Scietific Product), to prevent sample damage by the high intensity pump pulses. The path length is 129 μm, which is set by a Teflon spacer between two polished circular CaF 2 windows (25 × 2 mm, Koch Crystal Finishing). FTIR and UV–vis measurements FTIR and UV–vis measurements were made on 2 mM MG or MP solutions with various BSA concentrations (from 0 to 1 mM) held in DIR Amalgamated Sealed Cells (McCarthy Scientific) with a Teflon spacer (60 μm or 129 μm) between two polished rectangular CaF 2 windows (38.5 × 19.5 × 4 mm, Koch Crystal Finishing, Inc.). Steady state FTIR spectra were collected using a Varian 660 IR Spectrometer while steady state UV–vis spectra were collected using a Lambda35 Spectrophotometer (Perkin Elmer). How to cite this article: Li, G. et al . Anisotropic energy flow and allosteric ligand binding in albumin. Nat. Commun. 5:3100 doi: 10.1038/ncomms4100 (2014).